IKKβ regulates essential functions of the vascular endothelium through kinase-dependent and -independent pathways Vascular endothelium provides a selective barrier between the blood and tissues, participates in wound healing and angiogenesis, and regulates tissue recruitment of inflammatory cells. Nuclear factor (NF)-κB transcription factors are pivotal regulators of survival and inflammation, and have been suggested as potential therapeutic targets in cancer and inflammatory diseases. Here we show that mice lacking IKKβ, the primary kinase mediating NF-κB activation, are smaller than littermates and born at less than the expected Mendelian frequency in association with hypotrophic and hypovascular placentae. IKKβ-deleted endothelium manifests increased vascular permeability and reduced migration. Surprisingly, we find that these defects result from loss of kinase-independent effects of IKKβ on activation of the serine-threonine kinase, Akt. Together, these data demonstrate essential roles for IKKβ in regulating endothelial permeability and migration, as well as an unanticipated connection between IKKβ and Akt signalling. Nuclear factor (NF)-κB transcription factors (p65 or RelA, p50, p52, c-Rel, and RelB) generally exist as homo- or hetero-dimers in the cytosol bound to one of three inhibitory, IκB, subunits (reviewed in ref. 1 ). In response to a wide variety of stimuli, NF-κB is classically activated through serine phosphorylation and degradation of IκB via the ubiquitin pathway, followed by translocation of NF-κB to the nucleus where it activates transcription. Serine phosphorylation of IκB is mediated by a large multi-unit complex containing two catalytic subunits (I kappa B kinase (IKK)α and IKKβ) [2] , [3] , as well as the regulatory subunit IKKγ or NEMO [4] . IKKα has an important role in skin development independent of its kinase activity [5] as well as a specialized role in the alternative pathway of NF-κB activation that induces specific genes in B cells via NF-κB2 and RelB [6] . IKKβ appears to be the primary kinase mediating phosphorylation of IκB in most cell types and germline deletion of IKKβ results in embryonic lethality due to massive liver apoptosis [7] . In vascular endothelium, NF-κB activation is seen in a wide variety of diseases ranging from atherosclerosis [8] to cancer [1] . In addition to a role in endothelial inflammation, previous work has suggested a role for NF-κB in other essential endothelial functions. Pharmacological inhibition of NF-κB decreases vascular permeability [9] , although a recent report, using Tie2-driven transgenic overexpression of a superinhibitory IκB-α (sIκB), demonstrated increased vascular permeability after mustard oil stimulation as well as alterations in endothelial tight junctions [10] . Tie2-sIκB mice were born at the expected frequency and developed normally despite endothelial NF-κB inhibition [10] . A role in endothelial migration has not been reported, although IKKβ deletion promotes migration of embryonic fibroblasts [11] . To better delineate the role of IKKβ in mammalian endothelium in vivo , we used conditional inactivation to generate endothelial-specific IKKβ-deleted mice. These studies show essential roles for IKKβ in the developing placental and adult somatic vasculature, including regulation of endothelial apoptosis and migration, vascular permeability, and vasculogenesis. Surprisingly, although some of these effects (such as apoptosis) result from loss of IKKβ-kinase-dependent activation of NF-κB, others (such as permeability and migration) reflect loss of kinase-independent IKKβ modulation, the serine/threonine kinase, Akt. Together, these data demonstrate distinct kinase-dependent and -independent roles for IKKβ in regulating endothelial function, as well as an unanticipated connection between IKKβ and Akt signalling. Generation of endothelial-specific knockout mice To produce mice with endothelial deletion of IKKβ (IKKβ ΔEC ), we bred Tie2-Cre transgenic mice with IKKβ flox/flox mice [12] on an atherosclerosis-prone ApoE-null genetic background. Interestingly, Tie2-Cre + -IKKβ flox/flox -ApoE −/− mice were born at lower than the expected Mendelian frequency (7/48 versus 24/48 expected, P <0.0001 by chi-square analysis) raising the possibility of prenatal mortality and were ∼ 25% smaller than Cre-negative littermates at 8 and 32 weeks ( Fig. 1a , P <0.005 in repeated two-way ANOVA) in contrast to previously published results with Tie2-sIκB mice [10] . Collection of embryos after timed pregnancies revealed that 4/14 (29%) of the Tie2-Cre + -IKKβ flox/flox embryos on either an ApoE −/− or ApoE +/− were dead at E14–16 without evident gross malformation of major organs or vascular structures ( Fig. 1b ) compared with no fetal loss of the Tie2-Cre-negative IKKβ flox/flox embryos. Interestingly, placentae from embryos with endothelial IKKβ deletion were hypomorphic with fewer blood vessels ( Fig. 1c,d ). 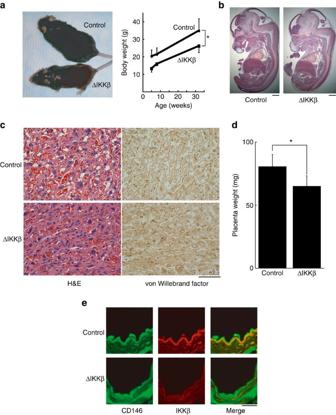Figure 1: Phenotype of endothelial-specific IKKβ knockout mice. (a) Photograph of littermate wild type ('control') and IKKβΔEC('ΔIKKβ') mice and body weight±s.d. shown from mice of each genotype at the indicated age (n=3/each group, *P<0.005 in repeated two-way ANOVA). (b) H&E staining of embryos at E14. Scale bars: 1 mm. (c) Staining of placentae by H&E and immunohistochemistry for von Willebrand Factor at E14. Scale bars: 10 μm. (d) Placenta weight from mice of each genotype (n=6 in IKKβΔECandn=3 in control mice, *P<0.05 in two-sided Student'st-test. Error bars:±s.d.). (e) Confocal microscopy images of vascular endothelium in IKKβΔECand control mice immunostained with antibody for CD146 and IKKβ. Scale bars: 100 μm. Figure 1: Phenotype of endothelial-specific IKKβ knockout mice. ( a ) Photograph of littermate wild type ('control') and IKKβ ΔEC ('ΔIKKβ') mice and body weight±s.d. shown from mice of each genotype at the indicated age ( n =3/each group, * P <0.005 in repeated two-way ANOVA). ( b ) H&E staining of embryos at E14. Scale bars: 1 mm. ( c ) Staining of placentae by H&E and immunohistochemistry for von Willebrand Factor at E14. Scale bars: 10 μm. ( d ) Placenta weight from mice of each genotype ( n =6 in IKKβ ΔEC and n =3 in control mice, * P <0.05 in two-sided Student's t -test. Error bars:±s.d.). ( e ) Confocal microscopy images of vascular endothelium in IKKβ ΔEC and control mice immunostained with antibody for CD146 and IKKβ. Scale bars: 100 μm. Full size image Intact vascular endothelium with altered function Intact vascular endothelium without detectable endothelial IKKβ expression in IKKβ ΔEC mice was demonstrated in confocal immunohistochemistry ( Fig. 1e ) and immunoperoxidase staining ( Supplementary Fig. S1a ) of mice after birth. Electron microscopy confirmed the presence of normal-appearing vascular endothelium, and, in contrast to results with transgenic overexpression of sIκB [10] , normal-appearing endothelial tight junctions ( Supplementary Fig. S1b–e ). To examine the structure and function of IKKβ ΔEC microvessels in vivo , we utilized in vivo microscopy of ear vessels after intravenous injection of Evans blue dye, which binds serum albumen ( Fig. 2a ; Supplementary Movie 1 ). Whereas vessel number and branching pattern appeared generally normal, dye rapidly extravasated in the endothelial IKKβ-knockout mice, indicating an increase in baseline vascular permeability even more severe than that seen in Tie2-sIκB mice [10] , as it occurred in the absence of stimulation and contrary to with the reduced permeability reported with pharmacological NF-κB inhibition [9] . 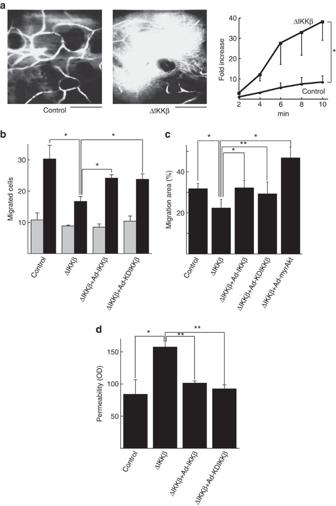Figure 2: Permeability and migration in IKKβ-manipulated endothelial cellsin vivoandin vitro. (a)In vivomicroscopy images of ear microvessels after injection of Evans blue dye. Representative image at 10 min (top) and cumulative data±s.e. from three independent experiments (bottom) are shown (*P<0.005 in repeated two-way ANOVA). Scale bars: 100 μm. See alsoSupplementary Movie 1online. (b)In vitromigration to VEGF of endothelial cells in which IKKβ is deleted or WT/-IKKβ is expressed. Cumulative data±s.e. from four independent experiments are shown. Grey bars: VEGF (−), black bars: VEGF (+). *P<0.05 in two-sided Student'st-test. (c) Wound-healing assay. Migration area was accumulated from six separated observation fields. Representative experiment is shown from three independent experiments total. *P<0.005 in two-sided Student'st-test. **P<0.05 in two-sided Student'st-test. Error bars: ±s.d. (d)In vitropermeability of endothelial cells in which IKKβ is deleted or WT/KD-IKKβ is expressed. Cumulative data±s.e. from three independent experiments are shown. *P<0.05 in two-sided Student'st-test. **P<0.005 in two-sided Student'st-test. OD, optical density. Figure 2: Permeability and migration in IKKβ-manipulated endothelial cells in vivo and in vitro . ( a ) In vivo microscopy images of ear microvessels after injection of Evans blue dye. Representative image at 10 min (top) and cumulative data±s.e. from three independent experiments (bottom) are shown (* P <0.005 in repeated two-way ANOVA). Scale bars: 100 μm. See also Supplementary Movie 1 online. ( b ) In vitro migration to VEGF of endothelial cells in which IKKβ is deleted or WT/-IKKβ is expressed. Cumulative data±s.e. from four independent experiments are shown. Grey bars: VEGF (−), black bars: VEGF (+). * P <0.05 in two-sided Student's t -test. ( c ) Wound-healing assay. Migration area was accumulated from six separated observation fields. Representative experiment is shown from three independent experiments total. * P <0.005 in two-sided Student's t -test. ** P <0.05 in two-sided Student's t -test. Error bars: ±s.d. ( d ) In vitro permeability of endothelial cells in which IKKβ is deleted or WT/KD-IKKβ is expressed. Cumulative data±s.e. from three independent experiments are shown. * P <0.05 in two-sided Student's t -test. ** P <0.005 in two-sided Student's t -test. OD, optical density. Full size image Another important function of vascular endothelium is cellular migration, which has a role in wound healing and angiogenesis. We measured the ability of IKKβ-deficient endothelial cells to migrate in response to the endothelial-specific stimulus, vascular endothelial growth factor (VEGF), in vitro . Endothelial cells from IKKβ flox/flox mice were infected with a Cre-expressing adenovirus, which effectively mediated deletion of IKKβ and inhibited NF-κB activation without affecting IKK-α or -γ ( Supplementary Fig. S2 ). Surprisingly, although IKKβ deletion enhanced fibroblast migration [11] , Cre-mediated deletion of IKKβ in endothelial cells cultured from IKKβ flox/flox mice reduced chemotactic migration to VEGF ( Fig. 2b ) and migration in a scratch wound-healing assay ( Fig. 2c ), suggesting a cell-specific role of IKKβ in regulating cell migration. Deletion of endothelial IKKβ ex vivo also recapitulated the increased permeability observed in vivo ( Fig. 2d ). Co-infection of endothelial cells with a recombinant adenovirus encoding wild-type IKKβ, but not a reporter construct, largely restored endothelial migration and reduced permeability to normal ( Fig. 2b–d ) demonstrating the specificity of this effect. Surprisingly, however, a kinase-inactive mutant of IKKβ (KD-IKKβ), which we had previously shown inhibits endothelial NF-κB activation [13] , also rescued these phenotypes with equal efficacy, suggesting they were not due to loss of kinase activity in the IKKβ null cells. Kinase assays confirmed that the wild-type IKKβ construct increased basal IKKβ kinase activity, which was further increased by cytokine stimulation ( Supplementary Fig. S3 ). In contrast, the KD-IKKβ construct did not manifest IKKβ kinase activity at baseline or in response to IL-1 stimulation ( Supplementary Fig. S3 ). Because NF-κB modulates cell survival through a variety of anti-apoptotic mechanisms [1] , we examined the effects of IKKβ deletion on apoptosis in endothelial cells. IKKβ deletion did not affect apoptosis in endothelial cells in the presence of serum but did result in a significant increase in apoptotic endothelial cells after serum deprivation ( Fig. 3 ). Expression of wild type (WT), but not KD IKKβ in IKKβ-deleted endothelial cells, mitigated serum starvation-induced apoptosis in endothelial cells ( Fig. 3 ). This result suggests that IKKβ has both kinase-independent and -dependent effects on important phenotypes of endothelial cells, and reinforces the specificity of results above for migration and permeability. 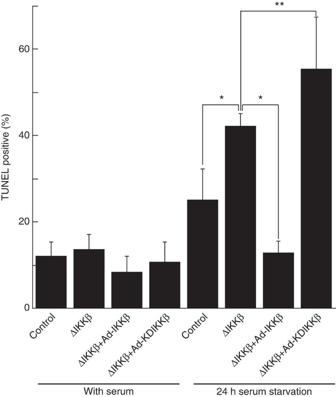Figure 3: Effect of IKKβ on apoptosis induced by 24 h serum starvation. Primary cultured endothelial cells from lungs of IKKβflox/floxmice with infection of Ad-GFP, Cre, IKKβ or KDIKKβ were serum-starved for 24 h. TUNEL positive cells were counted at seven independent fields (mean cell number: 241.5/field). *P<0.0005 in two-sided Student'st-test, **P<0.05 in two-sided Student'st-test. Error bars: ±s.d. Figure 3: Effect of IKKβ on apoptosis induced by 24 h serum starvation. Primary cultured endothelial cells from lungs of IKKβ flox/flox mice with infection of Ad-GFP, Cre, IKKβ or KDIKKβ were serum-starved for 24 h. TUNEL positive cells were counted at seven independent fields (mean cell number: 241.5/field). * P <0.0005 in two-sided Student's t -test, ** P <0.05 in two-sided Student's t -test. Error bars: ±s.d. Full size image Altered Akt signalling The abnormal growth and development as well as the severe vascular leakage seen in IKKβ ΔEC contrasted with results reported with endothelial NF-κB inhibition in Tie2-sIκB transgenics [10] , despite use of the same promoter. These differences in combination with kinase-independent rescue in vitro raised the possibility that IKKβ modulates baseline endothelial function through NF-κB-independent signalling pathways. Indeed, features of the IKKβ ΔEC mice were reminiscent of those seen in Akt1 null mice, including increased vascular permeability [14] and decreased endothelial migration ex vivo [14] , [15] , as well as prenatal mortality, hypotrophic and hypovascular placentae, and small size (thought in Akt1-null mice to reflect reduced Akt1-eNOS signalling in placental vascular endothelium [16] ). These similarities and previous reports that IKK isoforms (including IKKβ) [17] , [18] could physically interact with Akt prompted us to examine Akt in IKKβ ΔEC mice. Interestingly, phospho-Akt was markedly reduced in vascular endothelium from IKKβ ΔEC mice ( Fig. 4a ). Similarly, ex vivo deletion of IKKβ in endothelial cells resulted in reduced phosphorylation of Akt in response to insulin-like growth factor (IGF)-I ( Fig. 4b ). A similar blunted response to insulin was seen in IKKβ-deleted endothelial cells in vitro ( Supplementary Fig. S4 ). Phosphorylation of GSK3β in response to insulin was also blunted in IKKβ-deleted endothelial cells, consistent with inhibition of Akt downstream signalling ( Supplementary Fig. S5 ). Conversely, overexpression of either WT or kinase-inactive IKKβ in vitro was sufficient to increase Akt phosphorylation in endothelial cells ( Fig. 4c ), consistent with a kinase-independent effect of IKKβ on Akt signalling. Previous reports suggested that Akt and IKKβ physically interact in other cell types [18] . However, we did not find consistent evidence of robust IKKβ-Akt interaction despite multiple immunoprecipitation, GST-pull down and yeast interaction assays. 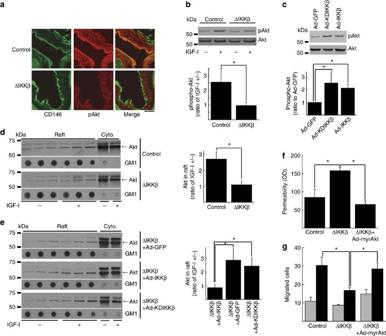Figure 4: Akt phosphorylation and localization in IKKβ-manipulated endothelial cellsin vivoandin vitro. (a) Confocal microscopy images of endothelial cells in IKKβΔECmice immunostained with antibody for CD146 and pAkt. Scale bar: 20 μm. (b) Representative immunoblots for pAkt and Akt in IKKβ-deleted endothelial cells treated with/without IGF-I and its cumulative quantitative densitometry data±s.d. from three independent experiments (*P<0.05 in two-sided Student'st-test). (c) Representative immunoblots for pAkt and Akt in endothelial cells overexpressed with WT- or KD-IKKβ and its cumulative quantitative densitometry data±s.d. from three independent experiments (*P<0.05 in two-sided Student'st-test). (d) Representative Akt immunoblots of fractions from sucrose gradient centrifugation of IKKβ-deleted endothelial cells treated with/without IGF-I and its cumulative quantitative densitometry data±s.e. from three independent experiments (*P<0.05 in two-sided Student'st-test). Ganglioside GM1 is marker for lipid raft fractions. (e) Representative Akt immunoblots of fractions from sucrose gradient centrifugation of IKKβ-deleted endothelial cells expressed with either WT- or KD-IKKβ treated with/without IGF-I and its cumulative quantitative densitometry data±s.e. (n=5 for ΔIKKβ+Ad-GFP;n=3 for ΔIKKβ+Ad-IKKβ;n=5 for ΔIKKβ+Ad-KDIKKβ; *P<0.05 in two-sided Student'st-test). Ganglioside GM1 is marker for lipid raft fractions. (f,g)In vitropermeability (f) and migration to VEGF (g) in endothelial cells in which IKKβ is deleted or myr-Akt is expressed. Gray bars: VEGF (−), black bars: VEGF (+) for (g). Each panel is cumulative data±s.e. from three independent experiments (*P<0.05 in two-sided Student'st-test). Figure 4: Akt phosphorylation and localization in IKKβ-manipulated endothelial cells in vivo and in vitro . ( a ) Confocal microscopy images of endothelial cells in IKKβ ΔEC mice immunostained with antibody for CD146 and pAkt. Scale bar: 20 μm. ( b ) Representative immunoblots for pAkt and Akt in IKKβ-deleted endothelial cells treated with/without IGF-I and its cumulative quantitative densitometry data±s.d. from three independent experiments (* P <0.05 in two-sided Student's t -test). ( c ) Representative immunoblots for pAkt and Akt in endothelial cells overexpressed with WT- or KD-IKKβ and its cumulative quantitative densitometry data±s.d. from three independent experiments (* P <0.05 in two-sided Student's t -test). ( d ) Representative Akt immunoblots of fractions from sucrose gradient centrifugation of IKKβ-deleted endothelial cells treated with/without IGF-I and its cumulative quantitative densitometry data±s.e. from three independent experiments (* P <0.05 in two-sided Student's t -test). Ganglioside GM1 is marker for lipid raft fractions. ( e ) Representative Akt immunoblots of fractions from sucrose gradient centrifugation of IKKβ-deleted endothelial cells expressed with either WT- or KD-IKKβ treated with/without IGF-I and its cumulative quantitative densitometry data±s.e. ( n =5 for ΔIKKβ+Ad-GFP; n =3 for ΔIKKβ+Ad-IKKβ; n =5 for ΔIKKβ+Ad-KDIKKβ; * P <0.05 in two-sided Student's t -test). Ganglioside GM1 is marker for lipid raft fractions. ( f , g ) In vitro permeability ( f ) and migration to VEGF ( g ) in endothelial cells in which IKKβ is deleted or myr-Akt is expressed. Gray bars: VEGF (−), black bars: VEGF (+) for ( g ). Each panel is cumulative data±s.e. from three independent experiments (* P <0.05 in two-sided Student's t -test). Full size image Disrupted Akt trafficking In response to growth factor stimulation, increased phosphatidylinositol (3,4,5)-trisphosphate (PIP3) binds the pleckstrin homology domain of Akt and prompts its translocation to the cell membrane, where it is localized in caveolar lipid rafts and phosphorylated, and subsequently moves to the nucleus [19] . Trafficking to lipid rafts has an important role in Akt activation [20] , and nuclear translocation enhances its anti-apoptotic effects [21] . IKKβ has also been reported to localize to lipid rafts [22] . To examine which step in the activation of Akt is affected by IKKβ deletion, we examined intracellular Akt trafficking after stimulation with IGF-I in murine endothelial cells in vitro . As previously described [19] , IGF-I stimulation of control cells induced early localization of Akt to the membrane (evident at 5 min) followed by movement to the nucleus (at 15 min) evident by confocal immunohistochemistry ( Supplementary Fig. S6a ). Subcellular localization of phosphorylated Akt followed a similar pattern ( Supplementary Fig. S6b ). In contrast, in endothelial cells in which IKKβ had been deleted, IGF-I-induced movement of both total and phospho-Akt to the cell membrane at 5 min and to the nucleus at 15 min were markedly inhibited ( Supplementary Fig. S6a and b ). Separation of membrane compartments on a sucrose gradient further documented that IKKβ deletion reduced Akt in membrane lipid raft fractions after IGF-I stimulation ( Fig. 4d ). Similarly, subsequent translocation of Akt to the nucleus after IGF-I treatment was inhibited by IKKβ deletion ( Supplementary Fig. S6c ). Importantly, endothelial caveolae are present in IKKβ ΔEC mice and appear normal by electron microscopy ( Supplementary Fig. S1b–e ), suggesting the observed changes in trafficking are not due to disruption of caveolae. Expression of either WT- or KD-IKKβ restored Akt trafficking to lipid rafts ( Fig. 4e ), consistent with the functional rescue of permeability and migration mediated by these constructs. Taken together, these data suggest that IKKβ deletion impairs Akt trafficking and subsequent activation and that the ability of IKKβ to enhance Akt localization to lipid rafts does not require IKK kinase activity. Akt rescues altered migration and permeability We tested the functional relevance of IKKβ's modulation of Akt activation in vitro . Of note, Chen et al . [14] previously demonstrated that permeability in Akt1-deficient endothelial cells is increased in a similar in vitro assay. As noted above, Cre-mediated deletion of IKKβ increased endothelial permeability and expression of either WT or KD IKKβ, which both restore Akt trafficking ( Fig. 4e ) and increase Akt phosphorylation ( Fig. 4c ), reduced endothelial permeability ( Fig. 2d ). Expression of activated Akt (myr-Akt) also restored permeability to normal in IKKβ-deleted endothelial cells ( Fig. 4f ). Similarly, expression of activated Akt (as well as either WT or KD IKKβ, Fig. 2b,c ) restored the ability of IKKβ-deleted endothelial cells to migrate in response to VEGF ( Fig. 4g ) and in a scratch wound-healing assay ( Fig. 2c ) in vitro . Together, these data suggest that deletion of IKKβ alters endothelial phenotype at least in part through kinase-independent regulation of Akt activation. Altered PTEN activity In the absence of evidence supporting a robust physical interaction between IKKβ and Akt, we examined the PTEN phosphatase, which cleaves PIP3, removing the primary stimulus for Akt translocation. Inhibitory phosphorylation of PTEN was significantly decreased by IKKβ deletion in endothelial cells, and conversely, overexpression of KD- or WT-IKKβ increased PTEN phosphorylation ( Fig. 5a–c ). These changes would be expected to increase PTEN phosphatase activity (and decrease Akt translocation/phosphorylation) after IKKβ deletion, and decrease PTEN phosphatase activity in a kinase-independent manner with overexpression. Direct measurement of PTEN phosphatase activity ( Fig. 5d ) confirmed that this was indeed the case. Taken together, these data implicate PTEN as a mediator of cross-talk between IKKβ and Akt, most likely through effects on the well-described pathway of PIP3-induced Akt membrane localization. 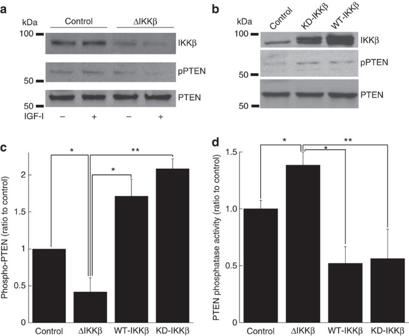Figure 5: PTEN phosphorylation and phosphatase activity in IKKβ-manipulated endothelial cells. (a–c) Representative immunoblots for IKKβ, pPTEN or PTEN in IKKβ-deleted endothelial cells (a) or WT/KD IKKβ expressed endothelial cells (b) and its cumulative quantitative densitometry data±s.d. from three independent experiments (c) (*P<0.05 in two-sided Student'st-test, **P<0.0005 in two-sided Student'st-test). (d) Phosphatase activity of PTEN in IKKβ-deleted or WT/KD IKKβ expressed endothelial cells. Cumulative data±s.d. from four independent experiments are shown (*P<0.005 in two-sided Student'st-test, **P<0.05 in two-sided Student'st-test). Figure 5: PTEN phosphorylation and phosphatase activity in IKKβ-manipulated endothelial cells. ( a – c ) Representative immunoblots for IKKβ, pPTEN or PTEN in IKKβ-deleted endothelial cells ( a ) or WT/KD IKKβ expressed endothelial cells ( b ) and its cumulative quantitative densitometry data±s.d. from three independent experiments ( c ) (* P <0.05 in two-sided Student's t -test, ** P <0.0005 in two-sided Student's t -test). ( d ) Phosphatase activity of PTEN in IKKβ-deleted or WT/KD IKKβ expressed endothelial cells. Cumulative data±s.d. from four independent experiments are shown (* P <0.005 in two-sided Student's t -test, ** P <0.05 in two-sided Student's t -test). Full size image Impaired ischemia-induced vasculogenesis The defect in VEGF-induced endothelial migration seen in vitro after IKKβ deletion raised the possibility that endothelial IKKβ would important in vasculogenesis or the formation of new blood vessels in adults. Given the small number of homozygous IKKβ ΔEC mice available for study, we addressed this question in heterozygous IKKβ ΔEC mice. After ligation of the common femoral artery, return of collateral flow was markedly impaired in heterozygous IKKβ ΔEC mice ( Fig. 6 ). These data are consistent with our in vitro observations and underscore the potential pathophysiological importance of endothelial IKKβ in vasculogenesis due to ischemia or potentially other stimuli. 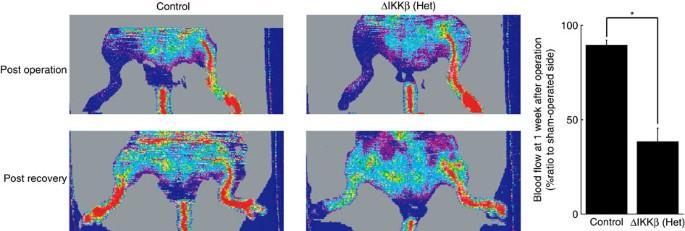Figure 6: Ischemia-induced neovascularizationin vivo. Representative images of blood flow after ligation of common femoral artery, and quantified cumulative data±s.d. from six animals (3 Cre-negative, 3 heterozygous IKKβΔECmice. *P<0.0005 in two-sided Student'st-test). Figure 6: Ischemia-induced neovascularization in vivo . Representative images of blood flow after ligation of common femoral artery, and quantified cumulative data±s.d. from six animals (3 Cre-negative, 3 heterozygous IKKβ ΔEC mice. * P <0.0005 in two-sided Student's t -test). Full size image To better delineate the role of IKKβ in mammalian endothelium, we used conditional inactivation to generate mice with endothelial-specific inaction of IKKβ (IKKβ ΔEC ). Gestational loss of IKKβ ΔEC embryos and stunted growth probably resulted from hypomorphic placentae. Late stage embryos and surviving adults manifested an intact somatic vasculature with surprisingly normal morphology. Loss of IKKβ blocked endothelial NF-κB activation. Whereas endothelial apoptosis was not increased at baseline, IKKβ-deleted endothelial cells were more susceptible to serum deprivation-induced apoptosis in vitro and apoptosis was mitigated by expression of wild-type but not kinase-inactive IKKβ. Adult animals lacking endothelial IKKβ manifest increased vascular permeability and impaired vasculogenesis in response to ischemia. In vitro , IKKβ-deleted endothelial cells also demonstrated increased permeability and reduced migration. Surprisingly, these defects were rescued equally well by wild-type and kinase-inactive IKKβ and appear related to kinase- independent activation by IKKβ of the serine/threonine kinase, Akt. Taken together, these data establish an important physiological role for IKKβ in regulating a variety of endothelial functions in mammals, and show unanticipated kinase-independent effects of IKKβ mediating cross-talk with Akt signalling. The increased vascular permeability seen in vivo in IKKβ ΔEC mice, is more severe than that seen with either isolated Akt1 deletion [14] or transgenic endothelial NF-κB inhibition [10] , probably reflecting the combined effects of endothelial inhibition of both Akt and IKKβ-NF-κB signalling. This inference is reinforced by the complex relationship of Akt signalling to endothelial permeability. Although Chen et al . [10] found increased permeability in Akt1 −/− endothelium both in vivo and in an in vitro model similar to the one used here, Ackah et al . [15] found reduced vascular permeability in Akt1 −/− mice in response to VEGF. These differences may reflect technical aspects of the assays used and/or the time-points examined. In addition, the IKKβ ΔEC mice studied here differ from the Akt1 −/− mice not only in the primary and concomitant loss of endothelial IKKβ signalling but also in that Akt signalling is preserved in non-endothelial cells, which may be an important source of a variety of factors affecting vascular permeability including VEGF and angiopoietins. Our data document cross-talk between two central signalling molecules, IKKβ and Akt, in endothelial cells in vitro and in vivo that appears mediated via the phosphatase, PTEN. Our results differ from previous reports in important respects. First, although we do find evidence of a signalling connection similar to that described previously [17] , [18] , [23] , here we find that Akt lies downstream of IKKβ (rather than the reverse), and the two molecules work together to exert important effects on baseline endothelial function. In addition, although it is difficult to completely exclude physical interaction as a contributor to these effects, our data suggest that PTEN has an important role as an intermediary. It is not clear whether these kinase-independent effects of IKKβ work via the IKK signalling complex. The observation that overexpression of IKKβ at levels nonstoichiometric to other components of the IKK complex increases Akt activation, raises the possibility that IKKβ acts independent of the complex in this context. In addition, we note that IKKα knockout mice [24] do not phenocopy any of the features we observed in IKKβ endothelial knockout mice, further supporting the hypothesis that IKKβ's role in this context does not require IKKα. However, testing these hypotheses awaits delineation of the precise molecular mechanism by which IKKβ modulates PTEN activity. In contrast to our results, several studies in other tissues have reported that IKKβ activation can inhibit insulin signalling in general and Akt in particular [20] , [25] , [26] . These differences may reflect tissue specific roles of IKKβ, similar to the skin-specific effects revealed by IKKα deletion [5] . However, even in other tissues, IKKβ-induced inhibition of Akt signalling was most pronounced in chronic inflammatory states or tissues with significant basal NF-κB activation [20] , [25] , [26] . The findings reported here occur in unactivated endothelial cells at baseline. As noted above, we also provide evidence of kinase-dependent effects of IKKβ on important endothelial phenotypes (for example, apoptosis), although not under basal conditions. Thus, it is quite possible that the relative importance of kinase-dependent and -independent IKKβ effects would shift, even in endothelial cells, in an inflammatory milieu. Nevertheless, these results broaden our understanding of the complex interactions of the IKK signalosome and demonstrate that IKKβ has important kinase- and NF-κB-independent effects, similar conceptually to those shown previously for IKKα [5] , in addition to its well-documented kinase-dependent effects. Most importantly, these data establish an essential role for IKKβ in fundamental endothelial functions including permeability and migration, and demonstrate the pathophysiological relevance of these effects in a model of ischemia-induced neovascularization. These findings and the observed interaction with Akt signalling may complicate efforts to target IKKβ in some diseases such as atherosclerosis but could be advantageous in other settings. For example, recent work suggests sustained endothelial Akt activation is necessary for maintenance of abnormal tumour vasculature [27] . As IKKβ is also a potential target for cancer therapy [1] , strategies aimed at decreasing IKKβ expression could provide additional benefit through secondary inhibition of endothelial Akt signalling and potentially through inhibition of angiogenesis. Understanding the role of IKKβ in vascular endothelium and the associated signalling cascades could help guide therapeutic strategies for a variety of conditions marked by endothelial activation and dysfunction. Antibodies and reagents Antibodies used include monoclonal anti-IKKβ (Upstate), polyclonal anti-IKKβ (H-470, Santa Cruz Biotechnology), anti-CD146 (Chemicon), anti-total and phospho-(Ser473)Akt, total and phospho-(Ser380/Thr382/383)PTEN, phospho-GSK3α/β (Cell Signaling). Catch & Release Immunoprecipitation kit (Upstate), ApopTag Red Apoptosis detection kit (Chemicon), NE-PER Nuclear and Cytoplasmic Extraction Reagents Kit (Pierce) and Cell Lysis Buffer (Cell Signaling ) were used in accordance with the manufacturers' instructions. Adenoviral vectors encoding WT IKKβ, kinase-defective (KD) IKKβ, myrAkt, EGFP, Cre and LacZ have been described previously in detail [13] , [28] . Animal studies All animal studies were performed after institutional approval and in compliance with applicable guidelines for animal experimentation. IKKβ flox/flox mice were mated with ApoE −/− (Jackson Immunoresearch Laboratories) to generate IKKβ flox/flox ApoE −/− mice which were mated with male Tie2-Cre mice to generate ultimately Tie2-Cre + -IKKβ flox/flox -ApoE −/− or Tie2-Cre + -IKKβ flox/flox -ApoE +/− mice. As the phenotype appeared identical on the ApoE −/− or +/− background, data from these mice was combined in some studies. Immunohistochemistry Slides were incubated in 80% acetone (2 min, 4 °C) and incubated in 3% hydrogen peroxide for 10 min. After incubation for 60 min, in blocking solution (5% goat serum, 5% donkey serum in tris buffered saline (TBS)), slides were incubated with diluted antibody for pAkt (1:50), polyclonal IKKβ (1:100) and CD146 (1:100) overnight at 4 °C. Diluted FITC-conjugated goat anti-mouse and rhodamine-conjugated donkey anti-rabbit secondary antibodies (Jackson, 1:100) were applied to the slides for 60 min. Immunoperoxidase staining Slides were incubated with Avidin Block (Vector Laboratories SP-2001, Avidin-Biotin blocking kit) for 15 min before applying Biotin Block for fifteen minutes. Diluted rabbit anti-Von Willibrand Factor (Chemicon, 1:200) was applied to each slide (4 °C, overnight). Diluted biotinylated donkey anti-rabbit secondary antibody (Jackson, 1:200) was applied for 60 min at room temperature. ABC reagent (Vector ) was applied to slides for 30 min at room temperature. DAB solution (diluted 1:10 in TBS, pH 7.6) added with 3% hydrogen peroxide (1:125) was applied to slides for approximately 1 min. Slides were then counterstained with hematoxylin. In vivo permeability assay Vessel permeability was assessed by leakage of the Evans blue dye from the mouse ear vasculature following intravenous injection. An intravenous catheter was inserted into the tail vein of anaesthetized mouse before placing the mouse on the stage of a video-rate scanning laser confocal microscope. The ear skin was gently spread onto a coverglass with a drop of 1% methocellulose. At the start of each experiment, 100 μl of 2% Evan's blue dye was injected via the tail vein. Images were acquired from an appropriate vascular area (at about 50 μm under the surface of the skin) and every 30 s for at least 10 min after injection. Each image was acquired by averaging 30 video frames (1 s integration time) using an Olympus 60×, numerical aperture 1.2, water-immersion objective producing optical sectioning images with sub-micron resolution comprising 500×500 pixels in a 300 μm×300 μm field of view. Evan's blue dye was excited by a 635 nm laser (Edmund Optics) and fluorescence detected through a 695±27.5 nm bandpass filter (Omega Optical) by a photo multiplier tube (Hamamatsu). To determine vessel permeability, acquired images (as a function of time) were first co-registered and then put in ImageJ as a stack. Using the polygonal selection tool, the change in fluorescence intensity was recorded in 4–8 tissues areas adjacent to blood vessel per stack. The fold increase of each transgenic animal ( n =3) was normalized to its littermate control at 2 min after injection and results were pooled. Endothelial cell culture Lungs of IKKβ flox/flox mice were harvested, minced finely and digested in 25 ml collagenase (Roche, 2 mg ml −1 ). Cells were incubated with anti-PECAM-1 antibody (BD Biosciences, 1:100) and cells bound with antibody were isolated magnetically with mouse anti-rat kappa microbead (Miltenyi Biotec), washed with complete media (DMEM, 20% FCS, 0.1 mg ml −1 heparin, 0.1 mg ml −1 endothelial cell mitogen (Biomedical Technologies), nonessential amino acids, sodium pyruvate, L -glutamine and penicillin/streptomycin at standard concentrations) and cultured in fibronectin-coated, tissue-culture flasks. Nonadherent cells were removed after 24 h and media replaced. At confluence, endothelial cells were magnetically selected further using anti-ICAM-2 antibody (BD Biosciences, 1:100). Endothelial migration assay Endothelial cells were suspended at 5×10 5 cells ml −1 and 100 μl were added to the top chamber of a fibronectin-coated transwell apparatus (6.5-mm diameter, 8-μm pore size Costar, Corning Incorporated) whose lower chamber was filled with 600 μl DMEM containing 50 ng ml −1 VEGF where indicated (Pepro Tech). Cells were incubated for 6 h at 37 °C in an atmosphere containing 5% CO 2 , and then fixed with ice-cold methanol for 20 min. Migrated cells were counted after staining with Hema3 Manual Staining System (Fisher Scientific) [29] . In vitro permeability assay Permeability assay was performed according to product manual (In vitro Vascular Permeability Assay from Millipore: ECM640). Endothelial cells monolayer forms on collagen-coated inserts which contain 1.0 μm symmetrical pores within a transparent polyethylene membrane. 150 μl of cell culture medium containing 1:40 FITC-Dextran is added on the top of the cells and incubated at 37 °C for three hours. The extent of permeability is determined by measuring the fluorescence of the plate well solution using excitation/emission wavelength of 485 nm/530 nm. Wound-healing assay Confluent endothelial monolayers in 6 cm dishes were scraped with sterilized 1 ml micropipette tips to create a cell-free zone. Microscopic images were captured at 0 and 36 h later, and the percent of the migrated area was quantified using Image J software (National Institutes of Health, USA). Sucrose gradient Endothelial cells were infected with the indicated adenoviral vectors, treated with 10 nM IGF-I or PBS for 15 min, and lysed in cell lysis buffer (Cell Signaling) containing 1 mM phenylmethylsulfonyl fluoride (PMSF). An identical amount of protein from each sample was mixed with 60% sucrose in PBS/MBS buffer 3 ml (final volume, sucrose concentration 51.7–58.7%), and transferred to a Beckman Ultracentrifuge tube. 3 ml of 35% sucrose followed by 4 ml of 5% sucrose were overlaid. Samples were ultracentrifuged (38,000 r.p.m. ≅ 180,000× g in SW41 rotor (Beckman Coulter), 20 h) and 24 fractions were collected from the top of the gradient. For detection of lipid raft fractions, all fractions were dot-blotted with HRP-labeled cholera toxin B (Sigma) to detect Ganglioside GM1, and raft fractions were immunoblotted for caveolin-1 (BD biosciences) for confirmation. PTEN activity assay PTEN activity assay was performed according to product manual (PTEN Activity Assay from Echelon: K-2300). Immunoprecipitated PTEN beads were washed with cell lysis buffer twice and with PTEN reaction buffer (10 mM Hepes, 150 mM NaCl, 10 mM DTT, ph 7.2) once, and re-suspended with 300 μl reaction buffer. 100 μl sample was added to each well of PI(3,4,5)P3-coated PTEN substrate plate, and plate was incubated for 90 min at 37 °C. Each well was washed with 200 μl of TBS-T three times, and PI(4,5)P2 detector was added to the well. Plate was incubated for 1 h at room temperature, and washed with 200 μl of TBS-T three times. 100 μl of HRP conjugate working solution prepared by diluting HRP conjugate 1:40 with TBS-GT was added to each well, and plate was incubated for 1 h at room temperature. After washing with 200 μl of TBS-T three times, 100 μl of TMB (Cell Signaling) was added to each well and plate was incubated for 30 min at room temperature. Reaction was stopped with 50 μl per well of stop solution (Cell Signaling) and absorbance was read at 450 nm. The values were compared with the standard curve to quantify conversion of PI(3,4,5)P3 substrate to PI(4,5)P2. Femoral artery ligation The epigastric and deep femoral arteries were cauterized. Proximal and distal sutures were placed around the femoral artery which was then cut between the ligatures. Immediately and one week after surgery, hindlimb blood flow was assessed using laser doppler imaging (LDI-2, Moor Inc). Flux, correlating to vascular limb perfusion, was quantitated using the Moor LDI-Main V51 software, and expressed as a ratio of the flux in the ischemic limb to that in the unoperated, nonischemic limb. Statistical analysis Unless otherwise specified in the text, statistical comparisons were made with two-sided Student's t -test. How to cite this article: Ashida, N. et al . IKKβ regulates essential functions of the vascular endothelium through kinase-dependent and -independent pathways. Nat. Commun. 2:318 doi: 10.1038/ncomms1317 (2011).